Unprecedented high-temperature CO2selectivity in N2-phobic nanoporous covalent organic polymers Post-combustion CO 2 capture and air separation are integral parts of the energy industry, although the available technologies remain inefficient, resulting in costly energy penalties. Here we report azo-bridged, nitrogen-rich, aromatic, water stable, nanoporous covalent organic polymers, which can be synthesized by catalyst-free direct coupling of aromatic nitro and amine moieties under basic conditions. Unlike other porous materials, azo-covalent organic polymers exhibit an unprecedented increase in CO 2 /N 2 selectivity with increasing temperature, reaching the highest value (288 at 323 K) reported to date. Here we observe that azo groups reject N 2 , thus making the framework N 2 -phobic. Monte Carlo simulations suggest that the origin of the N 2 phobicity of the azo-group is the entropic loss of N 2 gas molecules upon binding, although the adsorption is enthalpically favourable. Any gas separations that require the efficient exclusion of N 2 gas would do well to employ azo units in the sorbent chemistry. Nanoporous polymers [1] , [2] , [3] , [4] , [5] , [6] (pore width 1–100 nm) show considerable promise in gas capture [7] , storage [8] and separation technologies [9] , and as nano-filtration membranes [3] , catalysts [10] , drug delivery vehicles [11] and charge carriers [12] , [13] . These mostly organic polymers can easily be designed and constructed via facile synthetic protocols. To date, several crystalline and amorphous nanoporous organic materials with tunable functionality have been developed—namely, COF [14] , PIM [15] , HCP and CMP [16] , [17] , CTF [18] , PAF [19] , PPN [20] , POF [21] , BILP [22] , EOF [23] , PECONF [24] and COP [25] . CO 2 discharge into the atmosphere has risen with the increasing consumption of fossil fuels [3] , adversely affecting the fight against global warming [26] . CO 2 scrubbing by ethanolic aqueous amines [27] is yet to be challenged as a practical solution, despite the claims that numerous porous solids have better physicochemical properties and lower energy penalties [2] , [28] . In order to avoid energy-intensive CO 2 capture, we have to resort to physisorptive processes (enthalpy of adsorption, Q <40 kJ mol −1 ) rather than chemisorptive ones ( Q >40 kJ mol −1 ) (ref. 29 ). Physisorption, however, brings new challenges. First, there is the lack of CO 2 selectivity as there is no chemical bond being formed. Second, when the functional groups are tuned in order to enhance selectivity, CO 2 uptakes are hindered [30] . Third, no structure has been identified that rejects N 2 , a crucial but missing link in boosting CO 2 selectivity in post-combustion conditions. In this work, we introduce the concept of N 2 phobicity in order to achieve high CO 2 /N 2 selectivities without compromising CO 2 uptake. Our findings show an unprecedented increase in selectivity with increasing temperature, a previously unknown behaviour. To achieve this objective, we have synthesized a whole new class of nitrogen-rich nanoporous polymers, the azo-linked covalent organic polymers (azo-COPs) and found that their azo (–N=N–) groups reject N 2 gas selectively. Azo-COPs, with Brunauer–Emmett–Teller (BET) surface areas up to 729 m 2 g −1 , can store significant amount of CO 2 (up to 151.3 mg g −1 ) and show a very high CO 2 /N 2 selectivity (288) at 50 °C, an industrially relevant temperature (>40 °C). Azo-COPs are found to be extremely stable up to 350 °C in air as well as in boiling water for a week. A larger entropy loss associated with N 2 adsorption onto the azo groups of the framework as compared with CO 2 explains the high selectivity as well as its temperature dependence. This unique property of azo-COPs, along with their thermal and chemical stability, makes them ideal candidates for post-combustion CO 2 separations. Synthesis Azo compounds can be prepared by simple synthetic protocols [31] , where aromatic amines are oxidized using stoichiometric amounts of metal catalysts, resulting in the formation of desired products. Although effective, these methods are not sustainable and environmentally benign because of the need for rare or transition metals [32] . Here, we have followed a metal catalyst-free synthesis employing the direct coupling of a nitro aromatic compound, tetrakis(4-nitrophenyl)methane, A , and amines, 4,4′,4″,4′′′-methanetetrayltetraaniline, B1 , p -phenylenediamine, B2 , and benzidine, B3 , under basic conditions for the formation of interwoven, highly porous and amorphous aromatic azo-COPs ( Fig. 1 ). 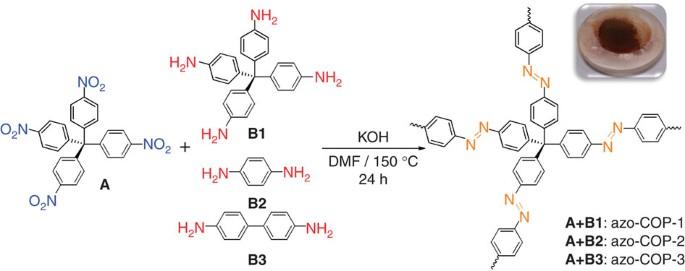Figure 1: Syntheses of a series of azo-COPs. Orange powders of azo-COPs were obtained by reacting tetrakis(4-nitrophenyl)methane,A, with three aromatic amines, namely 4,4′,4″,4′′′-methanetetrayltetraaniline (B1, azo-COP-1),p-phenylenediamine (B2, azo-COP-2) and benzidine (B3, azo-COP-3), in DMF at 150 °C in the presence of potassium hydroxide under an atmosphere of N2. Figure 1: Syntheses of a series of azo-COPs. Orange powders of azo-COPs were obtained by reacting tetrakis(4-nitrophenyl)methane, A , with three aromatic amines, namely 4,4′,4″,4′′′-methanetetrayltetraaniline ( B1 , azo-COP-1), p -phenylenediamine ( B2 , azo-COP-2) and benzidine ( B3 , azo-COP-3), in DMF at 150 °C in the presence of potassium hydroxide under an atmosphere of N 2 . Full size image Physicochemical characterizations The formation of azo-COPs was revealed by Fourier transform infrared spectroscopy (FTIR), elemental analysis, cross-polarization magic-angle spinning (CP/MAS) 13 C NMR and ultraviolet–visible spectroscopies ( Supplementary Figs S1–S3 ). The characteristic stretching band for –N=N– functionality in the FTIR spectrum is clearly visible at 1,447 and 1,403 cm −1 along with the respective bands for aromatic rings [33] . The FTIR bands located at 1,520 and 1,340 cm −1 correspond to N–O stretching mode, suggesting the presence of unreacted terminal nitro groups. The presence of terminal nitro groups is also evidenced by elemental analysis, which indicates the presence of oxygen in azo-COPs ( Supplementary methods section). In addition, the presence of bands in the range of 3,600–3,000 cm −1 indicates that there are terminal amino groups present in the structure. The presence of chemical shifts in CP/MAS 13 C NMR spectra of azo-COPs, namely, azo-COP-1, azo-COP-2 and azo-COP-3 (also named as COP-68, -69, -70), ( www.porouspolymers.com ) located at 150.2, 144.7, 129.5, 123.4 and 54.9 ppm confirmed the formation of the azo-linked aromatic polymers [19] , [34] . Azobenzene moieties have a characteristic ultraviolet–visible spectra where an intense absorption band at 360 nm indicates the presence of trans -azobenzene unit [35] . The solid-state ultraviolet–visible analysis revealed [34] that the as-synthesized azo-COPs have predominantly trans configuration and feature low band gaps ( Supplementary Figs S3, S4 ). Porous polymers are known [36] to be amorphous solids. Broad powder X-ray diffraction patterns of azo-COPs ( Supplementary Fig. S5 ) refer to their amorphous nature. Small-angle X-ray scattering analysis of azo-COPs, however, exhibited ( Supplementary Fig. S6 ) mesostructured character for azo-COP-1 and -2, whereas azo-COP-3 has a completely amorphous framework. The thermogravimetric analysis of azo-COPs ( Supplementary Fig. S7 ) indicate that they are stable up to 350 °C in air and 300 °C under N 2 environment. The mass losses can be assigned to desorption of trapped solvent molecules and the decomposition of the framework. It is well-known [25] that CO 2 scrubbing operations require high chemical stability as harsh conditions such as steam are employed frequently. In order to investigate the water stability of azo-COPs, we kept the polymers in boiling water for a week and measured their surface areas. Azo-COPs did not show any noticeable loss of surface area or CO 2 capacity ( Supplementary Fig. S8 ), indicating that network structures are highly robust. The bulk-scale morphology of azo-COPs was examined ( Supplementary Figs S9, S10 ) with field-emission scanning electron microscope and transmission electron microscope. Irregular-shaped particles of similar sizes are arranged to give a macroporous surface. The reasonably monodisperse grains are consistent with a homogeneous reaction, an essential feature for a large-scale industrial production. Azo-COP-2 has the smallest particles of all three, hence its enhanced gas sorption. Azo compounds feature low band gaps (for example, 2.22–2.35 eV for azo-COPs), evaluated from ultraviolet–visible diffuse reflectance spectroscopy ( Supplementary Fig. S4 ). Azo-bridged polymeric materials are also widely studied [37] for their optical storage applications. As optically stored information is only stable below glass transition temperature ( T g ), a high T g means more potential in optical data storage. All three azo-COPs show T g values of 158.6 °C ( Supplementary Fig. S11 ) in a differential scanning calorimetry (DSC) investigation, suggesting their potential for incorporation into optical storage devices. Argon physisorption measurements at 87 K were performed [38] ( Fig. 2 ) in order to evaluate the pore structure of the azo-COPs. We have shown that azo-COP-1, -2 and -3 are microporous and exhibit typical type-I reversible sorption profiles. The BET surface areas were found to be 635, 729 and 493 m 2 g −1 (BET linear plot, Supplementary Fig. S12 and Supplementary Table S1 ), and total pore volumes of 0.39, 0.44 and 0.32 cm 3 g −1 for azo-COP-1, azo-COP-2 and azo-COP-3, respectively. The pore width maxima of azo-COP-1, azo-COP-2 and azo-COP-3 centred at 0.7, 0.48 and 0.8 nm, respectively. The hysteresis at low pressures may be attributed to the pore networks effect [36] and also to the irreversible binding of gas molecules to the micropore surface. The calculated BET surface areas obtained from N 2 sorption isotherms of azo-COPs at 77 K ( Supplementary Figs S13, S14 ) commensurate with the ones from Argon physisorption measurements. The BET surface areas of azo-COPs were also measured using CO 2 as an adsorbate at 273 K (ref. 39 ), demonstrating surface areas of 303, 334 and 206 m 2 g −1 for azo-COP-1, azo-COP-2 and azo-COP-3, respectively ( Supplementary Fig. S15 ). 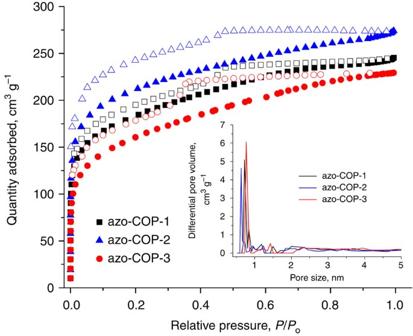Figure 2: Argon adsorption–desorption isotherms of azo-COPs at 87 K. Filled and empty symbols represent adsorption and desorption, respectively. For nitrogen isotherms at 77 K and BET linear plots of azo-COPs seeSupplementary Fig. S12. Inset: pore volume versus pore size. All the experiments were carried out using 1 g of each azo-COP. Figure 2: Argon adsorption–desorption isotherms of azo-COPs at 87 K. Filled and empty symbols represent adsorption and desorption, respectively. For nitrogen isotherms at 77 K and BET linear plots of azo-COPs see Supplementary Fig. S12 . Inset: pore volume versus pore size. All the experiments were carried out using 1 g of each azo-COP. Full size image Selective gas sorption CO 2 and N 2 are two apolar molecules with similar and small kinetic diameters, namely 3.30 and 3.64 Å (ref. 40 ), respectively. Their quadrupole moments (2.85 to 1) and polarizabilities (1.5 to 1), however, differ enough to design CO 2 -philic solids, which would be neutral towards N 2 . Owing to the presence of an electron-deficient carbon atom, CO 2 is expected to interact with protic electronegative functionalities (for example, amines) leading to a strong chemisorption, while N 2 remains impartial. So far, this simple interaction has led to a plethora of nanoporous polymers where the nitrogen-rich functionalities, such as triazine [1] , [18] , tetrazole [3] , imidazole [41] , phosphazene [24] , imide [42] and amines [25] , [43] , are built in. In all these and many other situations [2] , CO 2 -philicity is the main driving force for the CO 2 /N 2 selectivity, without taking into account any chemical architecture that would repel N 2 molecules selectively. The significance of the microporosity and the nitrogen-rich framework of azo-COPs have been investigated for their uptake of CO 2 and N 2 gas molecules. The CO 2 and N 2 adsorptions of the azo-COPs were measured up to 1 bar at 263, 273, 298 and 323 K in order to mimic post-combustion CO 2 capture conditions ( Fig. 3 , Table 1 ). Before the measurements, the azo-COPs were degassed at 150 °C for 5 h (see Methods) for both activation purposes and also to avoid any contribution from cis -azobenzene units. All the measurements were carried out using 1 g of azo-COPs to minimize errors associated with the mass of the adsorbents. The CO 2 isotherms are completely reversible and show an adsorption capacity of 145.4 mg g −1 for azo-COP-1, 151.3 mg g −1 for azo-COP-2 and 103.3 mg g −1 for azo-COP-3 at 263 K. This high affinity is a consequence of the favourable interactions of the polarizable CO 2 molecules through dipole–quadrupole interactions with the framework, and also the inherent microporosity of azo-COPs. At 273 K, CO 2 uptake is 107.6 mg g −1 for azo-COP-1, 112.4 mg g −1 for azo-COP-2 and 85.1 mg g −1 for azo-COP-3. As expected, the CO 2 uptake of azo-COPs decreases at 298 K, to 65.3 mg g −1 for azo-COP-1, 67.3 mg g −1 for azo-COP-2 and 53.6 mg g −1 for azo-COP-3. These values are still comparable to the very high surface area porous polymers [25] , such as PPN-4 (ref. 20 ) (65 mg g −1 ) and PAF-1 (ref. 19 ) (45 mg g −1 ). A smooth adsorption–desorption cycle implies that the interaction between CO 2 and the networks are weak enough to regenerate these azo-COPs without too much energy. Similar behaviour has been reported where adsorption on basic sites do not require heating to regenerate porous polymers [41] , [44] . The CO 2 isosteric heat of adsorption ( Q st ) is calculated from the adsorption data at 263, 273, 298 and 323 K [45] . The Q st for azo-COP-1, azo-COP-2 and azo-COP-3 are in the range of 24.8–32.1 kJ mol −1 , values which are comparable to those obtained with the previously reported [45] porous polymers. Slightly higher heats of adsorption are ascribed to the presence of –N=N– moieties in the framework of the azo-COPs. 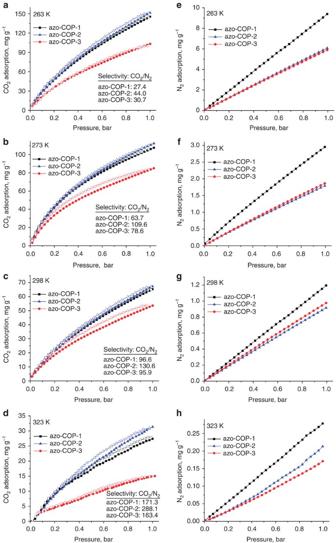Figure 3: CO2and N2adsorption–desorption isotherms of azo-COPs at different temperatures. CO2(a–d) and N2(e–h) gas isotherms measured up to 1 bar at 263, 273, 298, 323 K. Filled and empty symbols represent adsorption and desorption, respectively. Inset: respective CO2/N2selectivity. Increase in the CO2/N2selectivity with increasing temperature proves the N2phobicity of the framework while retaining its CO2-philic character. Figure 3: CO 2 and N 2 adsorption–desorption isotherms of azo-COPs at different temperatures. CO 2 ( a – d ) and N 2 ( e – h ) gas isotherms measured up to 1 bar at 263, 273, 298, 323 K. Filled and empty symbols represent adsorption and desorption, respectively. Inset: respective CO 2 /N 2 selectivity. Increase in the CO 2 /N 2 selectivity with increasing temperature proves the N 2 phobicity of the framework while retaining its CO 2 -philic character. Full size image Table 1 CO 2 and N 2 uptakes, selectivities and isosteric heat of adsorptions of azo-COPs. Full size table For a post-combustion CO 2 adsorption, CO 2 should be adsorbed preferentially over N 2 at high temperatures (>40 °C). To the best of our knowledge, however, all the porous polymers reported so far [2] , [41] , [44] exhibit significant loss in CO 2 /N 2 selectivity on going from 273 to 298 K ( Supplementary Table S2 ). Contrary to the common trend, azo-COPs show ( Table 1 ) higher CO 2 /N 2 selectivities with increasing temperatures. The selectivities were calculated using the Ideal Adsorbed Solution Theory (IAST) for CO 2 :N 2 mixture in the ratio of 0.15:0.85 ( Table 1 , Supplementary Figs S16–S20 ) and Henry's Law constants from the isotherms in the linear low pressure (<0.1 bar) range ( Supplementary Table S2 , Supplementary Figs S21–S23 ). The IAST CO 2 /N 2 selectivities of the azo-COPs range from 27.4 to 44.0 at 263 K, 63.7 to 109.6 at 273 K, 95.9 to 130.6 at 298 K and become 163.4 to 288.1 at 323 K, which is being the highest reported CO 2 /N 2 selectivity at 323 K to date. N 2 uptake drops ~70% at a temperature increase from 273 to 298 K, compared with a ~40% drop for CO 2 . This unprecedented behaviour cannot be explained only by conventional CO 2 affinities. A new concept, namely N 2 phobicity, is the result. When the CO 2 /N 2 selectivities found here are compared with those for other nitrogen-rich porous polymers ( Supplementary Table S2 ), azo-COPs show a lot less affinity towards N 2 . For example, covalent triazine-based frameworks (CTFs) reveal a mere CO 2 /N 2 selectivity of 31.2 at 273 K. Our earlier work on triazines [25] leads to the understanding [46] that an imidic bond (–C=N–) is not N 2 -phobic. Benzimidazole-linked polymers [41] show selectivities up to 113 at 273 K, being reduced to 71 at 298 K. Although nitrogen-rich organic cage frameworks [30] , [47] show high CO 2 /N 2 selectivities up to 213 at 298 K, their surface areas (<10 m 2 g − 1 ) and CO 2 capture capacities (up to 7.15 mg g −1 ) are very low. Other structures with protic nitrogens also behave in a similar fashion [43] , [44] , [48] . Computational studies As the aromatic rings present in the azo-COPs cannot be the reason for N 2 phobicity [19] , [20] , we studied the effects of the –N=N– moieties in the framework on the near rejection of N 2 at higher temperatures, 323 K, as well as the temperature dependence of the increased selectivity. Incidentally, similar observations have been noted in a very recent report [49] , where azo-bridged linkers are compared with ethylenic ones in crystalline metal-organic frameworks (MOFs) for CO 2 uptake. The authors, however, ignored the obvious N 2 -phobic behaviour of azo-MOFs when N 2 uptakes are compared. Under the same conditions (195 K), argon uptake follows a nonspecific interaction, thus serving as a control for the N 2 -phobic behaviour of the framework incorporating azo-bridged linkers. Our findings are commensurate with their data, in the sense that taken together, they prove the existence of N 2 phobicity. We first compared the relative binding affinity of the –N=N– group towards CO 2 versus N 2 using trans -azobenzene as a model system ( Fig. 4a ). The lowest energy structure of the CO 2 / trans -azobenzene complex indicates that CO 2 preferentially binds with the azo-group of trans -azobenzene with binding energy (BE) of 17.0 kJ mol −1 while N 2 preferentially binds to the phenyl-group with BE=11 kJ mol −1 , rather than to azo (BE=9 kJ mol −1 ). CO 2 also has a favourable interaction with aromatic ring involving large stabilization energy, 14.4 kJ mol −1 . As the experimental heat of adsorption for the present COPs observed for CO 2 is 25–32 kJ mol −1 ( Table 1 ), it appears that CO 2 interacts with more than one azo- or aromatic functionalities in COPs owing to the amorphous structural nature. Owing to a difficulty in structure prediction for the amorphous polymers [36] , we instead considered the coordination pillared-layer network (CPL-4) [50] , a closest crystalline MOF with azo moiety. Incidentally, our computed binding energies of the azo-group with CO 2 and N 2 are similar to the observed CO 2 and N 2 heats of adsorption [50] for CPL-4, -20 and -12 kJ mol −1 , respectively, where the multiple interactions with more than one functional group is not feasible owing to the structural rigidity of the MOFs. Of the two interaction moieties in the experimental azo-COPs, azo and aromatic rings, the azo-group is clearly the deciding factor for N 2 phobicity considering a large difference in azo-affinity for CO 2 versus N 2 (17.0 versus 9.0 kJ mol −1 ), while the phenyl ring has a relatively comparable binding affinity towards both CO 2 and N 2 , 14.4 and 11.0 kJ mol −1 , respectively. These results support the experimental trend that more azo-substitution increases the selectivity. The ab initio relative binding affinity for CO 2 versus N 2 (3–8 kJ mol −1 ) is in reasonable agreement with the experimental relative heat of adsorption data for various azo-COPs (5–9 kJ mol −1 ). Energy decomposition analysis [51] suggests that the frozen density repulsion as well as the lack of sufficient dispersion interactions between N 2 gas molecules and the azo groups are responsible for the moderate binding strength of N 2 /azo interaction compared with the stronger CO 2 /azo binding ( Supplementary Fig. S24 ). Despite the favourable heat of adsorption (−19.5 kJ mol −1 ), the fact that N 2 is nearly rejected, we can conclude that the rejection must have its origin in entropy. 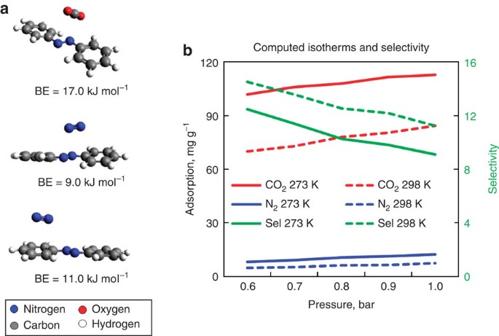Figure 4: Computational analysis for the gas affinity of azo linkages. (a) The RIMP2 minimum energy structures of CO2/trans-azobenzene and N2/trans-azobenzene complexes with the associated binding energies (BEs). (b) The computed isotherms for CO2(red) and N2(blue) obtained through GCMC simulation and the CO2/N2selectivity (green) at 273 K (solid line) and 298 K (dashed line). From this viewpoint, an upper bound of the adsorption entropy for N 2 might be estimated approximately as: Figure 4: Computational analysis for the gas affinity of azo linkages. ( a ) The RIMP2 minimum energy structures of CO 2 / trans -azobenzene and N 2 / trans -azobenzene complexes with the associated binding energies (BEs). ( b ) The computed isotherms for CO 2 (red) and N 2 (blue) obtained through GCMC simulation and the CO 2 /N 2 selectivity (green) at 273 K (solid line) and 298 K (dashed line). Full size image In order to understand the observed temperature dependence of the selectivity, we recall that the selectivity is related to Where Δ G ads is the free energy of adsorption and its temperature derivative is the entropy of adsorption (assuming constant heat capacity or enthalpy) In other words, the rate of increase in adsorption free energy with temperature is determined by the entropy change upon gas adsorption. As in usual enthalpy–entropy compensation, the higher BE (large negative Δ H ads ) would cause a tighter association with a corresponding loss in entropy (large negative Δ S ads ). Therefore, the conventional enthalpy–entropy compensation would predict ΔΔ G ads to increase (or selectivity to decrease) with temperature owing to a negative that is, , as in most previous temperature-dependent selectivity measurements [2] , [41] , [44] . However, the present azo-COPs show the opposite temperature dependence of the CO 2 /N 2 selectivity, suggesting positive ΔΔ S ads , that is, the entropy loss in the event of N 2 adsorption should be larger than that associated with the CO 2 adsorption ( Supplementary Fig. S25 ). In order to support this entropic origin qualitatively, we performed the grand canonical Monte Carlo (GCMC) simulations and analysed the trajectories on CPL-4. Figure 4b shows that the isotherms of CO 2 (red) and N 2 (blue), and the selectivity (green) at 273 (solid line) and 298 K (dashed line) within the pressure range between 0.6 and 1.0 bar. For convenience, we use the computed selectivity simply defined as the uptake ratios of different gases. As temperature rises, the gas uptakes decrease as expected; however, the selectivity increases (from solid to dashed lines) as in experiments. The interaction energy distribution between the gas and framework and the distance distribution between the centre of mass of the gas molecule and the centre of the azo-group are simulated at 263 K and 1.0 bar ( Supplementary Fig. S26 ). For both distributions in energy (0.6 versus 4.1 kJ mol −1 for N 2 versus CO 2 ) and configuration (0.48 versus 0.70 Å) space, the widths of distributions corresponding to the CO 2 binding with azo are much broader than those for N 2 . A similarly narrower distance distribution between N 2 and the aromatic ring (width being 0.50 Å) was also observed. No significant change in the energy distribution was observed with pressure up to 1 bar ( Supplementary Fig. S27 ), indicating that the binding sites are roughly the same regardless of the loading. The narrower distance distributions obtained for N 2 binding qualitatively suggest that azo–N 2 interactions have configuration space that is much less accessible for binding than the case of CO 2 , which makes the adsorbed N 2 retain lower (more unfavourable) entropy than the adsorbed CO 2 . The net effect is then positive ΔΔ S ads , leading to negative temperature dependence in , or increased selectivity with temperature. We note, however, that our interpretation assumes constant (or weak) temperature dependence for enthalpy of adsorption for CO 2 and N 2 , which needs to be further investigated. We have evolved a catalyst-free synthesis of robust, N 2 -phobic, nanoporous azo-COPs with surface areas up to 729 m 2 g −1 . These azo-COPs reveal carbon dioxide uptake twice as much as the industrial standard, monoethanolamine, while the selectivity for carbon dioxide over nitrogen is 288 at 50 °C. The increased selectivity for carbon dioxide over nitrogen, as well as the thermal and water stability of the azo-COPs at industrially relevant temperatures, suggests potential applications for these materials in post-combustion carbon dioxide capture and in air separations. It is not unlikely that these N 2 -phobic azo-COPs will provide design principles for the development of next-generation porous polymers for highly selective gas separations, such as natural gas purification. Looking into the broader picture, CO 2 -related gas separations require the following four fundamental guidelines for the proposed adsorbent materials: (1) water stability [29] , (2) selectivity [3] , (3) thermal stability [1] and (4) cost [25] . Any newly discovered sorbent candidate has to be evaluated for all these prospects. Not to mention, studying temperatures <40 °C usually mislead in identifying the best sorbent as both pre-combustion and post-combustion processes run at warmer temperatures. Synthesis of azo-COPs-1,2,3 All reagents and solvents employed in the synthesis were commercially available and used as received without further purification. In a typical synthesis, orange powders of azo-COPs were obtained in 40–57% yields by reacting tetrakis(4-nitrophenyl)methane with aromatic amines—for example, benzidine, p -phenylenediamine, 4,4′,4′′,4′′′-methanetetrayltetraaniline—in DMF in the presence of KOH under an inert atmosphere of N 2 , where the reaction temperature was raised to 150 °C and stirred for 24 h. Once completed, the reaction was cooled to room temperature and stirred in an excess of distilled water for 1 h. The precipitate was filtered off and washed with warm distilled water ( × 4), followed by washing with Me 2 CO ( × 3) and THF ( × 3). Subsequently, an orange precipitate was dried at 110 °C under vacuum for 4 h. All the azo-COPs were reproducible on multigram scales. The synthesis of monomers and detailed synthetic routes for azo-COPs are provided in the Supplementary methods section. Characterization methods FTIR spectra were recorded on KBr pellets using a Perkin-Elmer FTIR spectrometer. Solid-state CP/MAS 13 C NMR spectra of azo-COPs were collected by a Bruker Avance III 400 WB NMR spectrometer. Liquid 1 H and 13 C NMR spectra were taken using DMSO-d 6 as the solvent in a 400 MHz Bruker NMR spectrometer. Thermogravimetric analysis was performed on a NETZSCH-TG 209 F3 instrument by heating the samples to 800 °C at a rate of 10 °C min −1 under air and N 2 atmospheres. DSC of azo-COPs was measured by NETZSCH DSC 204 F1 instrument (Germany) at a scan rate of 10 °C min −1 in a nitrogen flow in the range of −60 to +280 °C. X-ray diffraction patterns of the samples were acquired from 2 to 70° by a Rigaku D/MAX-2500 (18 kW) micro-area X-ray diffractometer. Small-angle X-ray scattering data for powdered azo-COPs were obtained on a Rigaku D/MAX-2500 diffractometer. The morphology of azo-COPs was studied by field emission scanning electron microscopy on a Philips XL30SFEG instrument. TEM images were collected by field emission transmission electron microscope (200 KV, Tecnai F20). Samples for TEM investigations were prepared by putting an aliquot of alcoholic dispersion of azo-COPs onto an amorphous carbon substrate supported on a copper grid. The excess liquid was then removed, and the grid was allowed to dry at room temperature. The absorbance spectra of azo-COPs were collected on a ultraviolet–visible spectrophotometer where the powder samples were sandwiched between two quartz glasses and irradiated by a 365-nm ultraviolet lamp (8 W; 230 V; ~50/60 Hz from Vilber Lourmat, France) . In order to evaluate the porosity of azo-COPs, Ar and N 2 adsorption isotherms were obtained with a Micromeritics ASAP 2020-accelerated surface area and porosimetry analyser at 87 and 77 K, respectively, after the samples had been degassed at 150 °C for 5 h under vacuum. The adsorption–desorption isotherms (Ar at 87 K and N 2 at 77 K) were obtained to give the pore parameters, including BET ( P / P o =0.01–0.25) and Langmuir ( P / P o =0.1–0.35) surface area, pore size and pore volume. The pore size distribution of azo-COPs was calculated from the Ar and N 2 adsorption isotherms by the Non-Local Density Functional Theory method using a cylindrical pore model. IAST data were calculated using OriginPro v8.5 ( Supplementary methods section). Pore volume of azo-COPs was calculated at P / P o=0.95. The low-pressure CO 2 and N 2 adsorption–desorption isotherms for azo-COPs were measured at 263, 273, 298 and 323 K using a static volumetric system (ASAP 2020, Micromeritics Inc., USA). The temperature during adsorption and desorption was kept constant using a circulator. Before the adsorption measurements, the samples were dried at 110 °C for 24 h. The samples were further activated in situ by increasing the temperature at a heating rate of 1 K min −1 up to 423 K under vacuum (5 × 10 −3 mm Hg) and the temperature and vacuum was maintained for 5 h before taking the sorption measurements. All the adsorption–desorption experiments were carried out twice to ensure the reproducibility. There were no noticeable differences in the isotherm points obtained from both experiments. Heats of adsorption were determined from CO 2 and N 2 adsorption isotherms at 263, 273, 298 and 323 K using a Micromeritics ASAP 2020 instrument and the standard calculation routines in the Datamaster offline data reduction software (Micromeritics). Computational details Quantum chemical calculations for the binding energies of CO 2 – and N 2 – trans -azobenzene complex and their energy decomposition analysis were performed using Q-CHEM [52] . To describe nonbonding interactions between the framework and gas molecules correctly, we used the RIMP2/VDZ(d) geometry optimizations, and the final binding energies were further refined with the complete basis set limit using the RIMP2/aug-cc-pV(DT)Z extrapolation. The isotherms and equilibrium ensembles for the CO 2 and N 2 uptakes in the CPL-4 frame containing the azo-group were obtained using GCMC simulations with the Cerius2 v4.0 software. The force field parameters and charges for CO 2 were adopted from Harris et al. [53] —Dreiding 2.21 and equilibrium charge method. How to cite this article: Patel, H.A. et al . Unprecedented high-temperature CO 2 selectivity in N 2 -phobic nanoporous covalent organic polymers. Nat. Commun. 4:1357 doi: 10.1038/ncomms2359 (2013).